Observation of Landau levels in potassium-intercalated graphite under a zero magnetic field The charge carriers in graphene are massless Dirac fermions and exhibit a relativistic Landau-level quantization in a magnetic field. Recently, it has been reported that, without any external magnetic field, quantized energy levels have been also observed from strained graphene nanobubbles on a platinum surface, which were attributed to the Landau levels of massless Dirac fermions in graphene formed by a strain-induced pseudomagnetic field. Here we show the generation of the Landau levels of massless Dirac fermions on a partially potassium-intercalated graphite surface without applying external magnetic field. Landau levels of massless Dirac fermions indicate the graphene character in partially potassium-intercalated graphite. The generation of the Landau levels is ascribed to a vector potential induced by the perturbation of nearest-neighbour hopping, which may originate from a strain or a gradient of on-site potentials at the perimeters of potassium-free domains. The charge carriers in graphene are known to follow a relativistic Dirac equation and behave as massless Dirac fermions (DFs) [1] . In a magnetic field, massless DFs in graphene exhibit a relativistic Landau level (LL) quantization and an anomalous quantum Hall effect [2] , [3] . The LL energy sequence in graphene (single layer) shows a square-root dependence on both the magnetic field and the Landau index n , where a zeroth LL appears at the Dirac point. However, it has been reported recently that, without any external magnetic field, quantized energy levels have been observed in the density of states of highly strained graphene nanobubbles on a platinum (111) surface by scanning tunnelling spectroscopy (STS). These quantized peaks were attributed to the LLs of massless DFs in graphene formed by a strain-induced pseudomagnetic field [4] . Alkali metal-graphite intercalation compounds (GICs) have been extensively investigated for their layered geometric and electronic structures, where charge transfer from alkali metals to graphite π * and interlayer bands takes place [5] , [6] , [7] , [8] , [9] . Intercalated alkali metal atoms are known to form a domain structure called the Daumas–Herold domain, which is distributed within graphite to comprise a stage structure [10] , [11] . In GICs, the layer–layer interaction has been reported to be significantly weaker than the strong intra-layer interaction and the π -character is maintained in the carbon layer [5] . Recently, a study of KC 8 (stage-1 of potassium-intercalated graphite) by angle-resolved photoemission spectroscopy (ARPES) has indicated that the interlayer coupling of KC 8 is negligible and that a linear dispersion relation of the π and π* bands is observed in the low-energy region of the band structure [12] . The linear dispersion was attributed to the generation of DFs of graphene. Owing to the appearance of the graphene character by alkali metal intercalation into graphite, the local electronic properties of GICs, which may provide new insights into the understanding of GICs and graphene, become of great interest. In this study, a partially potassium-intercalated highly oriented pyrolytic graphite (K-HOPG) sample was prepared and the local electronic structure at the atomic level was examined with scanning tunnelling microscopy (STM) and STS. Here we report the generation of the LLs of massless DFs on the K-HOPG surface in the absence of an external magnetic field. The pseudomagnetic field is estimated to be as much as 251 T. The observation of the LLs of massless DFs indicates appearance of the graphene character in K-HOPG. The generation of the LLs is ascribed to a vector potential induced by the perturbation of nearest-neighbour (NN) hopping, which may originate from a strain or a gradient of on-site potentials at the perimeters of potassium-free domains. Corrugated surface due to K-free domains in K-HOPG The K-HOPG sample was prepared by depositing potassium on a HOPG surface at room temperature in an ultra-high vacuum chamber. After deposition, the HOPG sample was heated to approximately 800 K to desorb the surface potassium. A typical STM image of the K-HOPG surface is shown in Fig. 1a . The image shows irregularly shaped dark regions, which are not observed on clean graphite surfaces (see also Supplementary Fig. S1 ). The STM image obtained with an atomic resolution ( Fig. 1b ) shows that the ordered atomic arrangement is continuous on the surface with only a slight twist at the boundary between the bright and dark regions. More clearly, the line profile across the boundary ( Fig. 1c ) reveals a continuous slope with a periodicity of the atomic arrangement, indicating that the top layer of graphite is intact with corrugation at the boundaries. Generally, an STM image reflects not only the geometric structure but also the density of states [13] . 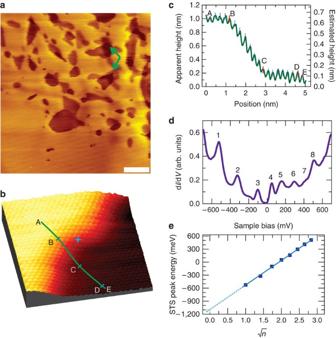Figure 1: Corrugated surface of K-HOPG and STS spectra therein showing Landau levels. (a) STM topography in large-scale, constant-current mode (−100 mV, 2.0 nA, 315×336 nm2). The green arrows indicate the overlapping of dark patterns. The white scale bar is 53 nm. (b) STM topography at the boundary of a dark pattern (−100 mV, 320 pA, 6.28×6.72 nm2). (c) Line profile of the green line inbshowing continuous height modulation across a boundary. (d) STS obtained at a boundary indicated by the blue star inb. (e) Linear scaling between the peak positions in the STS and. Error bar is below ±20 meV in each case. We thus estimated the real height by analysing the STM image, as shown in Figure 1c . The details of the analysis are described in Supplementary Methods and Supplementary Fig. S2 . The bright region was found to be higher than the dark region by 0.53–0.60 nm, which is smaller than the apparent height. The sizes of the dark regions typically range from 8 to several tens of nanometres wide and from 0.2 to 0.6 nm deep. In addition, the contrast in the STM image is independent of the polarity of the bias voltage ranging from −300 to +300 mV. In other words, the contrast mainly corresponds to the height modulation and the intact top carbon layer is corrugated. The Rutherford backscattering result of K-HOPG shows that K is intercalated in the bulk and diffused into deep layers ( Supplementary Fig. S3 ). Similar patterned STM images have been reported for a lithium-intercalated graphite surface, where the patterns in the image were also attributed to partial intercalation [14] . The graphene layer–layer distance is known to increase when alkali metal atoms are intercalated [5] . In the present study, the bright and the dark regions observed in the STM image are considered to correspond to the potassium-intercalated regions and the potassium-free domains, respectively. This consideration is consistent with the STS results and density functional theory (DFT) calculations, as is described below. Thus, many valleys of the potassium-free domains can be regarded as being distributed inhomogeneously. Figure 1: Corrugated surface of K-HOPG and STS spectra therein showing Landau levels. ( a ) STM topography in large-scale, constant-current mode (−100 mV, 2.0 nA, 315×336 nm 2 ). The green arrows indicate the overlapping of dark patterns. The white scale bar is 53 nm. ( b ) STM topography at the boundary of a dark pattern (−100 mV, 320 pA, 6.28×6.72 nm 2 ). ( c ) Line profile of the green line in b showing continuous height modulation across a boundary. ( d ) STS obtained at a boundary indicated by the blue star in b . ( e ) Linear scaling between the peak positions in the STS and . Error bar is below ±20 meV in each case. Full size image It should be noted that the darkness within the dark regions in the STM image is also inhomogeneous, showing the overlap of dark regions (green arrows in Fig. 1a ; Supplementary Fig. S4 ). This inhomogeneity can be explained by the overlapping of nanovalleys in different carbon layers. The overlapped dark regions are frequently observed, indicating that the nanovalleys in different layers tend to overlap with each other ( Fig. 1a ; Supplementary Fig. S4 ). This can be explained by the alternative interlayer interaction between the K δ+ domain and the negatively doped graphene. As a result, potassium-free domains tend to be overlapped. The corrugated surface was formed spontaneously; the contribution of scanning-induced migration to pattern formation is negligible, because the corrugated patterns were observed even at the beginning of the STM measurements. Meanwhile, the shapes of the dark regions in the STM image changed slightly during the long-time scanning at 4.6 K (several hours), owing either to scanning-induced migration or to thermal diffusion (see Supplementary Fig. S4 ). LLs of DFs in K-HOPG without magnetic field The local density of states near the Fermi level ( E F ) at the perimeter of a dark region (blue star in Fig. 1b ) of the K-HOPG surface was measured by STS ( Fig. 1d ). Eight distinct peaks appear in the region between −700 and +700 mV in the STS spectrum. These quantized levels are similar to the LLs observed for two-dimensional materials in a magnetic field [15] , where the energies of the quantized LLs follow a specific relationship with the quantum number (Landau index, n ), that is, the energies of the LLs follow the linear relationship with n , or , in the case of normal two-dimensional electronic systems (2DES), bilayer graphene and graphene, respectively [16] . By examining the energy of each peak as a linear function of the Landau index n , , and, , we found a best fitting (Pearson's r is 0.9993) in the linear relationship between the peak energy and ( Fig. 1e ) when the first peak from the left (−525.5 mV) is assigned to LL n =1. The detailed analysis process is summarized in Supplementary Methods and Supplementary Fig. S5 . The relationship of massless DFs in a magnetic field is expressed as where E n is the energy of the n th LL with respect to E F , E Dirac is the energy of the Dirac point (DP), ω c is the cyclotron resonance frequency due to the magnetic field B , e is the electron charge, ħ is Planck's constant divided by 2π and ν F is the Fermi velocity [1] , [2] , [3] . The appearance of the monolayer graphene character is comparable to the linear dispersion measured for KC 8 by ARPES, indicating negligible interlayer coupling [12] . According to equation (1), the LL at n =0 (LL 0 ) is located at the DP, independent of the strength of the magnetic field. By extrapolating the linear relationship between E n and ( Fig. 1e ), the energy of the DP was estimated to be −1.11 eV with respect to E F . The DP shift, which is attributed to the charge transfer from potassium to graphite, was comparable with that for KC 8 (−1.35 eV) as measured by ARPES [12] . A shift in the DP has also been reported for a potassium-adsorbed graphene surface on SiC based on an ARPES study, wherein the DP gradually shifted to lower energies with increasing amounts of potassium and finally shifted to approximately −0.7 eV when the doping amount reaches 0.0350 electron per unit cell [17] . The density of potassium near the HOPG surface in the present study is considered to be relatively high, because the significant DP shift in this study is close to that measured for KC 8 . That is, potassium-intercalated regions are dominant on the surface, consistent with the suggestion that the dominant bright regions in the STM image ( Fig. 1a ) correspond to the potassium-intercalated regions. LLs were, in fact, frequently observed near the perimeters of the dark regions ( Fig. 2 ; Supplementary Fig. S6 ). 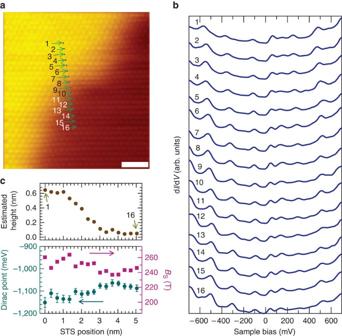Figure 2: Electronic structures across a boundary with derived Dirac points and pseudomagnetic fields. (a) STM topography at the boundary (−100 mV, 320 pA, 6.28×6.72 nm2). The white scale bar is 1.1 nm. (b) STS spectra obtained simultaneously with the STM at the position indicated ina. (c) The estimated heights at the STS measuring positions ina(upper panel). The Dirac points and pseudomagnetic fields (BS) at the STS measuring positions inaderived from the STS spectrab(lower panel). The error bars indicate standard deviations. Figure 2a,b shows the STS results obtained at different positions across the boundary region. All 16 STS spectra exhibited the same character as that shown in Fig. 1d (the same as no. 8 in Fig. 2b ), with quantized states in the spectra for both the bright and dark regions ( Fig. 2b ). All the STS results could be fitted linearly to in the same manner as shown in Fig. 1e (see Supplementary Fig. S7 ), and the estimated DPs from each fit are shown in Fig. 2c . The DPs in the bright and dark regions are −1.14 and −1.08 eV, respectively, that is, there is a difference of 60 meV between the DP energies from the bright and dark regions. In other words, the DPs for the bright region are located lower from E F than those for the dark region. It is considered that the difference in DP energy corresponds to that between potentials for K δ+ -intercalated and K δ+ -free regions close to the boundary. In the K δ+ -intercalated region, the Coulomb potential of K δ+ is screened by locally high density of electrons, that is, the screening effect [18] , which causes the small difference in potential (60 meV) between K δ+ -intercalated and K δ+ -free regions close to the boundary. It is possible that LLs feel the difference in potential. Figure 2: Electronic structures across a boundary with derived Dirac points and pseudomagnetic fields. ( a ) STM topography at the boundary (−100 mV, 320 pA, 6.28×6.72 nm 2 ). The white scale bar is 1.1 nm. ( b ) STS spectra obtained simultaneously with the STM at the position indicated in a . ( c ) The estimated heights at the STS measuring positions in a (upper panel). The Dirac points and pseudomagnetic fields ( B S ) at the STS measuring positions in a derived from the STS spectra b (lower panel). The error bars indicate standard deviations. Full size image Here, it should be noted that the STS in Fig. 1d has an apparent parabolic background with the LLs, showing symmetrically band-like features of the π and π* states on both sides of E F . This background cannot be attributed to electron–phonon coupling-assisted tunnelling, because phonon-assisted tunnelling should give rise to a sharp feature at ±63 meV but not a broad background [19] . The parabolic background was assigned to the π and π* states for the subsurface graphitic layer or potassium-free domain. In fact, different types of electronic structures were observed by STS for the K-HOPG surface, such as band gap and parabolic graphite structures ( Supplementary Fig. S8 ). The electronic structure of graphite (parabolic structure in STS) was often observed inside the dark regions and the band gap structure was often observed for the bright regions far from the boundary. The observation of each kind of spectrum always depends on the measurement position but is independent of the observation sequence. Note that the parabolic π and π* states are not shifted in energy from E F , which is in contrast to the DP shift in the LLs. The inhomogeneous character implies that the electronic structure of graphite is locally modified by the intercalated K δ+ . In general, LLs appear in response to an external magnetic field. Although no external magnetic field was applied in this study, LLs appeared for the K-HOPG surface ( Fig. 1d ). The strength of the corresponding magnetic field can be estimated from the linear relationship between the LLs and (equation (1)). First, the cyclotron resonance frequency ω c was derived from the slope of the fitted line of E n versus . Next, the value of B was determined to be 251 T from the cyclotron resonance and using a Fermi velocity of 1.0×10 6 m s −1 . The derived values of B at different positions across the boundary region are plotted in Fig. 2c as B S , showing a high-magnetic field ranging from 236 to 264 T across the boundary. The estimated magnetic field is much stronger than that currently known for the strongest magnet (the Fermi velocity should be renormalized in doped graphene [20] , which would lead to estimation of a stronger pseudomagnetic field). Note that the estimated B S exhibits a position dependence anti-phase with that of the DP shown in Fig. 2c and Supplementary Fig. S6i , suggesting that a heavier doping (lower potential, potassium-intercalated region) leads to a higher magnetic field. Theoretically, the pseudomagnetic field in graphene induced by structural symmetry breaking has been predicted with a tight-binding approach [1] . It has been reported that inequivalent hopping between NN (different sublattice) induces a pseudomagnetic field in the tight-binding model [21] , [22] , [23] , [24] , [25] , [26] , in which perturbations in the hybridization of the NN atoms lead to a vector potential of an effective gauge field, and the modulation of the gauge field further leads to the generation of a pseudomagnetic field. Geometric disorders in graphene, such as curvature and/or strain, have been theoretically proposed to result in the perturbation of hopping [21] , [22] , [23] , [24] , [25] , [26] . The LLs observed in this study for K-HOPG in the absence of an external magnetic field can be thus attributed to the pseudomagnetic field originated from inequivalent hopping. Two models can explain the inequivalent hopping due to the partial intercalation of potassium. One attributes the inequivalent hopping to geometry disorders including strain and corrugation in the K-HOPG surface. The other assigns the cause to a gradient of the on-site potential at the perimeter of the potassium-free domain. To examine the two models, DFT calculations were carried out for a bilayer graphene partially intercalated with potassium. As shown in Fig. 3a–c , the calculated interlayer distances of the potassium-free and the potassium-intercalated regions were 0.344 and 0.558 nm, which are in agreement with those for graphite (0.335 nm) and KC 8 (0.535 nm) [5] , respectively. Thus, the difference in the calculated interlayer distances between the potassium-free and potassium-intercalated regions is 0.21 nm, which is smaller than that observed in our STM image (0.53 nm). The relatively large actual depth is explained by the overlapping of the dark regions (potassium-free domains) in the K-HOPG sample. Thus nanovalleys with different depths are thought to be formed at potassium-free domains, similar to the nanobubbles of graphene formed on Pt with heights of 0.3–2.0 nm in terms of the nanodomain feature. The strain formed at the perimeters of the nanovalleys may produce the LLs owing to geometric-disorder-induced hopping perturbation in the graphene layer, as described above [21] , [22] , [23] , [24] , [25] , [26] . However, bending of the graphene layer in K-HOPG is relatively smooth compared with the large curvatures of the nanobubbles (apex), although the strengths of their pseudomagnetic fields are comparable. For this reason, we propose another model to explain the high pseudomagnetic field, in which the difference in the on-site potential at the domain perimeter induces inequivalent hopping. In the DFT calculations, the on-site potentials of the carbon atoms differ by 0.6 eV between potassium-intercalated and potassium-free regions, and a potential gradient can be observed at the boundary ( Fig. 3d ). Equipotential contours should be produced near/along the perimeter of the potassium-free domain, leading to equivalent hopping in a contour. On the other hand, a potential gradient will form in the direction towards the centre of the potassium-free domain and leads to a hopping, which is inequivalent with that along the contour direction. The character at the perimeter of the potassium-free domains is similar to that for nanobubbles on Pt, because hopping in the contours of the nanobubbles is equivalent, whereas the hopping towards the apex is inequivalent with that along the contour direction. We currently consider both the strain and on-site potential to contribute more or less to the formation of the LLs. 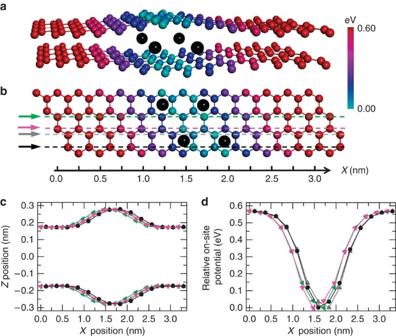Figure 3: Structure and on-site potential of partially potassium-intercalated bilayer graphene calculated by DFT. (a,b) A perspective side view and an orthogonal top view, respectively. The colour indicates the relative on-site potential of each carbon atom. The minimum energy is set as 0 eV. (c,d) TheZpositions and relative on-site potentials of the carbon atoms along the dashed lines inbwith the same colours as a function of theXposition, respectively. Figure 3: Structure and on-site potential of partially potassium-intercalated bilayer graphene calculated by DFT. ( a , b ) A perspective side view and an orthogonal top view, respectively. The colour indicates the relative on-site potential of each carbon atom. The minimum energy is set as 0 eV. ( c , d ) The Z positions and relative on-site potentials of the carbon atoms along the dashed lines in b with the same colours as a function of the X position, respectively. Full size image Preparation of K-HOPG A clean HOPG surface (ZYA grade, PGX 04, Panasonic) was prepared by cleavage in an air atmosphere followed by thorough degassing under ultra-high vacuum conditions; the clean surface was confirmed via low-temperature STM. The potassium was deposited by passing a current through a potassium dispenser placed above the HOPG surface at room temperature under ultra-high vacuum conditions. It is well known that potassium intercalation occurs spontaneously when the temperature is higher than 193 K [27] . To achieve effective intercalation by considering the diffusion process, the sample was left to stand at room temperature for 1 h and then annealed to 800±30 K for 5 min. STM and STS measurements STM investigations (USM-1500, UNISOKU) were performed at low temperature (4.6 K) in the constant-current mode by using a commercial Pt/Ir tip and standard lock-in techniques. Differential conductance spectra (STS) were obtained simultaneously during the STM measurements by instantly turning off the feedback loop and pausing the scan at the location of the predefined positions in the STM region. DFT calculations All calculations were performed on the basis of DFT. To express the exchange correlation energy among the interacting electrons, local density approximation was applied with a functional form fitted to a Monte-Carlo result for homogeneous electron gases [28] , [29] . Ultrasoft pseudopotentials were adopted to describe the electron–ion interactions [30] . The valence wave functions and charge density were expanded in terms of a plane-wave basis set with cut-off energies of 25 and 225 Ry, respectively. Brillouin-zone integration was carried out using a (1×4) k -mesh for performing both geometry optimization and self-consistent electronic structure calculations. Geometry optimization was performed for all atoms in the slab until the remaining force acting on the atoms was less than 0.005 Ry Å −1 . A conjugated-gradient minimization scheme was used for both electronic structure calculation and the geometry optimization. How to cite this article: Guo, D. et al . Observation of Landau levels in potassium-intercalated graphite under a zero magnetic field. Nat. Commun. 3:1068 doi: 10.1038/ncomms2072 (2012).